Size-dependent surface phase change of lithium iron phosphate during carbon coating Carbon coating is a simple, effective and common technique for improving the conductivity of active materials in lithium ion batteries. However, carbon coating provides a strong reducing atmosphere and many factors remain unclear concerning the interface nature and underlying interaction mechanism that occurs between carbon and the active materials. Here, we present a size-dependent surface phase change occurring in lithium iron phosphate during the carbon coating process. Intriguingly, nanoscale particles exhibit an extremely high stability during the carbon coating process, whereas microscale particles display a direct visualization of surface phase changes occurring at the interface at elevated temperatures. Our findings provide a comprehensive understanding of the effect of particle size during carbon coating and the interface interaction that occurs on carbon-coated battery material—allowing for further improvement in materials synthesis and manufacturing processes for advanced battery materials. Carbon coating is particularly effective for improving conductivity and surface chemistry in specific cathode materials used in lithium ion batteries (LIBs). For example, lithium iron phosphate (LFP) is a promising cathode material with superior stability but its performance is hindered by low electronic conductivity of 10 −9 S cm −1 (refs 1 , 2 , 3 ); however, an increase of five to eight orders of magnitude in electronic conductivity can be achieved with the use of carbon coating [4] , [5] , [6] , [7] . Since the first carbon-coating process on LFP was reported by Ravet et al . [8] , [9] , numerous studies have been dedicated to understanding the effects of this process [10] , [11] , [12] , [13] . During carbon coating, the carbon source produces a reducing atmosphere to protect Fe(II) from oxidation at elevated temperatures while simultaneously stabilizing the iron in LFP by hindering its transformation to metallic iron [9] . Despite significant achievements, a number of issues related to the reducing environment of carbon still remain unclear, including surface/interface reactions that occur between carbon and LFP [14] ; the formation of secondary phases [15] , [16] ; phase equilibrium [17] ; lithium volatility [6] ; and more importantly, the effect of LFP particle size on these surface/interface reactions [18] , [19] , [20] , [21] . To answer these questions, a suitable model for LFP material and tools to directly observe the surface/interface reaction are needed. In recent years, the melt-casting process is proposed as a method of choice for the production of industrial class LFP. Ingot LFP has a large flat surface and provides an ideal model to directly study the surface chemistry that occurs during the carbon-coating process [22] , [23] , [24] , [25] . With the ingot sample design, some basic information such as the interface chemistry reaction that occurs between carbon and LiFePO 4 during carbon coating can be obtained. In this work, LFP ingot material and commercial powder samples are used to demonstrate the direct visualization of a size-dependent surface phase-change process that occurs during the carbon-coating process. Furthermore, this surface phase change can be extended to both micro-sized and larger powder-based LFP materials. Unlike the instability behaviours commonly found in other nanomaterials under high temperatures, in this study, nano-LFP exhibits an extremely high stability during carbon coating. This unusual finding leads to further investigation towards the nature of the interface interaction that occurs between carbon and the underlying material as well as verify the importance of nanosized LFP—consideration of the purity and stability of the material when carbon coating is applied. Surface new-phase formation The most intriguing phenomenon is illustrated in Fig. 1 . Many ‘island-shaped’ phases (that is, bright colours) are observed on the surface of carbon-coated LFP ingot at 800 °C. These phases clearly arise from the substrate material and were given the name ‘top phase’—so that they may be distinguished from the underlying phase of the substrate. A close-up view outlined in Fig. 1a–d indicates the top phase material consisting of distinguished sharp edges and corners along with the occurrence of a striped pattern. These striped regions range in width from ~100 to 250 nm, and exhibit a three-dimensionally (3D) stripe-structured phase. The island shapes and associated morphological information indicates the formation of a secondary phase. The formation of 3D islands are due to a lattice mismatch-induced stress occurring at the material interface between two phases. During the carbon-coating process, this lattice mismatch stress drives the phase in the form of 3D islands on top of the remaining LFP layer—similar to previous results that mismatch strain evokes the creation of crystal islands [26] , [27] , [28] . We propose that these surface changes are directly related to the introduction of carbon or the carbon-coating process, as this phenomenon is not observed under H 2 -reducing or Ar atmospheric conditions, where carbon is absent ( Supplementary Information ). 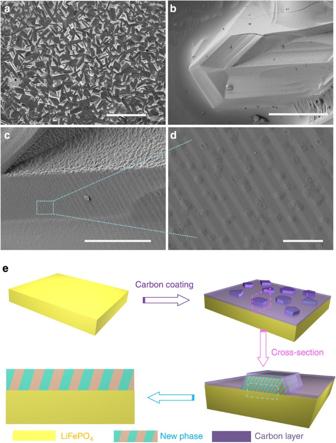Figure 1: Surface new-phase formation. (a–d) SEM image of surface phase formation on LiFePO4after carbon coating. (e) Schematic representation of surface phase formation on LiFePO4. Scale bar, 1 mm (a), 500 μm (b), 100 μm (c) and 1 μm (d). Figure 1: Surface new-phase formation. ( a – d ) SEM image of surface phase formation on LiFePO 4 after carbon coating. ( e ) Schematic representation of surface phase formation on LiFePO 4 . Scale bar, 1 mm ( a ), 500 μm ( b ), 100 μm ( c ) and 1 μm ( d ). Full size image Characterization of surface new phase Two sample slices—one from the top and the other from the bottom—with a thickness of 50~100 nm were obtained with the use of a focus ion beam (FIB) for observation under a HRTEM ( Supplementary Fig. 1 ). The top sample ( Fig. 2a ) shows uniform stripes and is consistent with scanning electron microscope (SEM) observations previously mentioned. A uniform carbon layer with a thickness of ~4 nm was also found to coat the surface of the sample (see Fig. 2b and insert in Fig. 2a ). Selected Area Electron Diffractions (SAED) in Fig. 2b indicate that the top sample is a new phase corresponding to Fe 2 P 2 O 7 ( Supplementary Fig. 2 ). In contrast, the bottom phase remains unaltered with no evidence of stripes ( Fig. 2c ), and is accompanied by a thicker carbon layer (8~10 nm) ( Fig. 2d ; Supplementary Fig. 3 ). SAED indicates that this bottom phase remains as LFP. It is evident that carbon coating leads to a surface phase change to occur on flat ingot sample material with the formation of a new secondary phase consistent with Fe 2 P 2 O 7 (top sample). 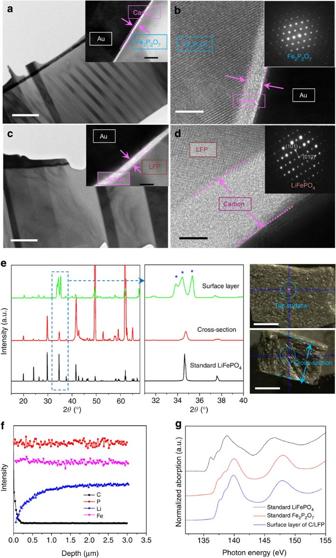Figure 2: Characterization of surface new phase. (a–d) HRTEM characterization of the top sample (a,b) and bottom sample (c,d). (e) Micro X-ray diffraction (μXRD) patterns and optical images of carbon-coated LiFePO4ingot at top surface and fresh-cut cross-section. (f) Dynamic secondary ion mass spectrometry (SIMS) profile of C, P, Li and Fe at carbon-coated LiFePO4ingot. (g) FLY of P L3,2-edge XANES spectra of Fe2P2O7, LiFePO4, and C/LiFePO4ingot. Scale bar, 1 μm (a,c), 20 nm the insert in panelsaandc, 5 nm (b,d) and 5 mm (e). Figure 2: Characterization of surface new phase. ( a – d ) HRTEM characterization of the top sample ( a , b ) and bottom sample ( c , d ). ( e ) Micro X-ray diffraction (μXRD) patterns and optical images of carbon-coated LiFePO 4 ingot at top surface and fresh-cut cross-section. ( f ) Dynamic secondary ion mass spectrometry (SIMS) profile of C, P, Li and Fe at carbon-coated LiFePO 4 ingot. ( g ) FLY of P L 3,2 -edge XANES spectra of Fe 2 P 2 O 7 , LiFePO 4 , and C/LiFePO 4 ingot. Scale bar, 1 μm ( a , c ), 20 nm the insert in panels a and c , 5 nm ( b , d ) and 5 mm ( e ). Full size image Micron X-ray diffraction (μ-XRD) was utilized on the carbon-coated sample with the use of two alternate methods—a top view for surface phase analysis and a fresh-cut cross-section for bottom phase identification ( Fig. 2e ). X-ray patterns of the coated sample surface indicate a large amount of secondary phase Fe 2 P 2 O 7 , whereas the bulk material inside remains as pure LFP. This data further confirms that a phase change occurs only on the sample surface. In contrast, there are no obvious secondary phases found in the XRD pattern for the Ar-annealed sample without carbon precursor additions. The lithium loss and formation of Fe 2 P 2 O 7 was also confirmed by dynamic secondary ion mass spectrometry and P L 3 , 2 -edge X-ray Absorption Near Edge Structure (XANES) spectra [29] , as shown in Fig. 2f,g . Synchrotron hard X-ray nano-tomography of surface new phase The new lithium deficient phase, Fe 2 P 2 O 7, was also identified with synchrotron hard X-ray full-field spectroscopic imaging and nano-tomography ( Fig. 3 ). The experiment was carried out at X8C beamline [30] at the National Synchrotron Light Source, Brookhaven National Laboratory. A cylindrical volume of interest was extracted from the surface of C/LiFePO 4 using focused ion beam and lifted-out using micro-manipulation ( Fig. 3a,b ). The presence of two different phases was confirmed with Fe 2 P 2 O 7 observed as white (higher X-ray attenuation) at the top of the sample and LiFePO 4 being grey at the bottom ( Fig. 3c ). Two-dimensional chemical mapping ( Fig. 3d ) and Fe K-edge XANES profile shown across the phase boundary ( Fig. 3e ) verify the presence of a new phase occurring on the surface of LiFePO 4 . Three-dimensional tomography was carried out at an X-ray energy of 7,120 eV, where the new phase and LiFePO 4 show a distinctive contrast in the Fe K-edge XANES. 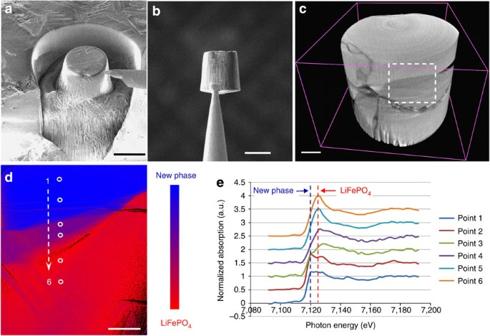Figure 3: Synchrotron hard X-ray nano-tomography of surface new phase. (a,b) FIB milling process at the surface of C/LiFePO4ingot sample. (c) The 3D morphology of the FIB sample. (d) The 2D chemical mapping of selected zone (white dashed box) at the FIB sample. (e) Fe K-edge of XANES profile of selected points ind. Scale bar, 20 μm (a,b), 5 μm (c) and 2 μm (d). Figure 3: Synchrotron hard X-ray nano-tomography of surface new phase. ( a , b ) FIB milling process at the surface of C/LiFePO 4 ingot sample. ( c ) The 3D morphology of the FIB sample. ( d ) The 2D chemical mapping of selected zone (white dashed box) at the FIB sample. ( e ) Fe K-edge of XANES profile of selected points in d . Scale bar, 20 μm ( a , b ), 5 μm ( c ) and 2 μm ( d ). Full size image In situ carbon-coating experiment and XRD analysis We further extended our study to powder-based LFP samples to further validate this interesting phenomenon. Powder-based LFP samples with different sizes (0.5–1 mm, 1–5 μm, 200–500 nm) were obtained by ball milling the above ingot sample. On close inspection of the surface phase-change process, carbon coating was directly observed on powder-based LFP (micron-sized grade, 1~5 μm, Phostech) by in situ SEM observations combined with injection of carbon precursor (ethylene) at 800 °C ( Fig. 4a ; Supplementary Movie 1 ). After coating, particle aggregation, shrinkage and surface melting, similar surface phases, form on the surface of LFP ( Fig. 4a ). During this process, a particularly violent surface-boiling reaction takes place on the larger-sized LFP particles ( Supplementary Movie 2 ). However, following carbon coating, nano-LFP (200–500 nm) shows negligible surface change as well as limited particle aggregation, even under prolonged coating conditions (1 h) ( Fig. 4b ; Supplementary Fig. 4 , Supplementary Movie 3 ). XRD analysis in Fig. 5a confirms that the new phase only appears with larger LFP samples (1–5 μm, 0.5–1 mm). The size-dependent surface phase change is related to LFP size effect on the carbon decomposition/precipitation process. Coated carbon thickness increases with smaller LFP particle size, as hydrocarbons are readily decomposed on nano-LFP due to enhanced catalytic effects ( Supplementary Fig. 5 ) [31] . 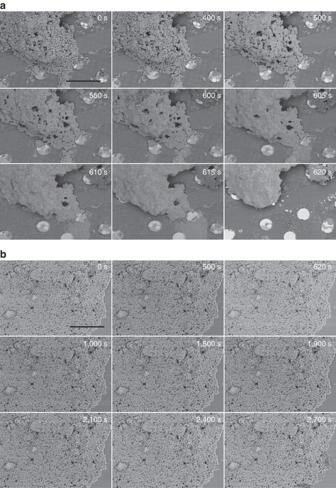Figure 4:In situcarbon-coating experiment. SEM observation on large-sized (a) and small-sized (b) LiFePO4powder. Scale bar, 20 μm (a,b). Figure 4: In situ carbon-coating experiment. SEM observation on large-sized ( a ) and small-sized ( b ) LiFePO 4 powder. Scale bar, 20 μm ( a , b ). 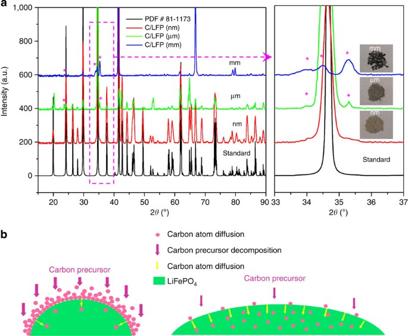Figure 5: New-phase formation at powder-based LiFePO4during carbon coating. (a) Micro X-ray diffraction (μXRD) patterns of carbon-coated LiFePO4with different sizes. (b) A schematic illustration of carbon-competitive diffusion/deposition at different-sized LiFePO4. Full size image Figure 5: New-phase formation at powder-based LiFePO 4 during carbon coating. ( a ) Micro X-ray diffraction (μXRD) patterns of carbon-coated LiFePO 4 with different sizes. ( b ) A schematic illustration of carbon-competitive diffusion/deposition at different-sized LiFePO 4 . Full size image The formation of new phases was previously reported by Zaghib et al . [32] However, new phases of nanosized γ-Fe 2 O 3 clusters were observed for non-carbon-coated LiFePO 4 , whereas ferromagnetic clusters do not exist in the carbon-coated LiFePO 4 (ref. 32 ). During the carbon-coating process, carbon does not penetrate LiFePO 4 but rather coats the particle surface. The deposited carbon may result in the reduction of Fe 3+ , preventing the formation of a ferromagnetic phase. By comparison, an alternate phase and mechanism is observed in our study that may result from the use of different sample size (ranging from nanometres to millimetres) for LiFePO 4 . Clearly, in our work, carbon coating has an essential role in surface phase change. Supplementary Fig. 6 shows the evolution of surface phase change with carbon coating over time, with increased surface morphology change occurring and larger island-like phases forming. Moreover, the surface phase change is independent of carbon precursor choice with similar changes occurring with various carbon precursors sources ( Supplementary Fig. 7 ). Similar to the decrease in melting point seen for metal and metal oxide materials after carbon introduction, the existence of carbon also decreases the melting point of LFP ingot due to solid solution behaviour. This results in a surface molten process for flat LFP, which is confirmed by the sample being fused to ceramic crucible holder following the carbon-coating process. The decrease in melting point for various metals and metal oxide materials in the presence of carbon has been previously demonstrated [33] , [34] . Under the similar conditions, the melting point of Fe 2 P 2 O 7 is also decreased by carbon coating, although it is theoretically close to 1,200 °C (ref. 35 ). During this molten process, the volatile and light element, lithium is evaporated in the form of Li 2 O under the following reaction mechanism: These phase changes occur readily under moderate reducing environments produced by carbon coating—resulting in a nonstoichiometric mixture existing in the molten phase. During the cooling process, a second phase of Fe 2 P 2 O 7 precipitates from the nonstoichiometric molten mixture as a result of Li 2 O loss. These surface phase change occurs under a broad temperature range ( Supplementary Fig. 8 ) and begin to occur at temperatures as low as 650 °C ( Supplementary Fig. 9 ). Our observations are also consistent with results reported by Zaghib et al . [36] who designed in situ HRTEM experiments to study the synthesis conditions of C/LiFePO 4 for use in LIBs. Their report indicates a structural destruction of LiFePO 4 accompanied by the production of unwanted secondary phases occurring at temperatures over 750 °C. Furthermore, heating LiFePO 4 to temperatures greater than 800 °C, results in its decomposition. Temperatures lower than 700 °C are not sufficient for the formation of crystalline LiFePO 4 and also produces an uneven carbon-coating layer. Therefore, 700 °C is suggested as the optimum synthesis temperature for the production of crystalline LiFePO 4 with a homogenous uniform carbon-coating layer. However, their report did not outline in detail the influence of particle size on carbon coating for LiFePO 4 . The formation of carbon coating on LFP involves a process of decomposition, deposition and diffusion ( Fig. 5b ). Following decomposition of carbon precursor, a competitive process ensues between the diffusion of carbon atoms into the crystalline lattice of LFP and aggregation of carbon atoms on the LFP surface. For LFP ingot and larger-sized samples (over several micrometres), hydrocarbon decomposition occurs relatively slowly, resulting in active carbon atoms rapidly submerging into the crystalline lattice of LFP by diffusion before aggregating on the ingot surface. Once the carbon concentration within the LFP reaches a critical value, the melting point of LFP is decreased and the ingot surface melts to form a C/LFP molten alloy. The decrease in melting point and continuous interaction between hydrocarbon and LFP contributes to surface melting, resulting in a molten state and subsequent surface phase reactions occurring. The volatilization of Li 2 O and/or CO 2 and CO from decomposition of carbon precursor forms pockets of gas—as observed in the boiling phenomenon seen under SEM ( Supplementary Movie 2 ). The loss of lithium in large-sized LFP samples was also confirmed by inductively coupled plasma atomic emission spectroscopy (ICP-AES) testing ( Supplementary Tables 1 and 2 ). For nano-LFP particles, however, hydrocarbon decomposition occurs rapidly due to the elevated catalytic effects, resulting in elevated carbon concentration being generated on the particle surface. Furthermore, the precipitation rate of carbon atoms on the surface of nano-LFP is much higher than the diffusion rate of carbon atoms into LFP and a solid carbon layer readily encloses the particle surface before the carbon concentration in the crystal has a chance to reache the critical value required for particle melting. Once nano-LFP is covered with a thick layer of carbon, its catalytic effect ceases and the hydrocarbon decomposition rate decreases substantially—protecting the LFP surface chemistry and limiting the interaction between LFP and hydrocarbon. Thus, nano-LFP exhibits extremely high stability during carbon coating. In summary, we have shown that a size-dependent surface phase change occurs in LFP during the carbon-coating process. This surface phase change is visible at temperatures as low as 650 °C, which approximates industrial processing temperatures. Our findings show that efforts to achieve a high volumetric energy density for C/LFP through micro and larger-size processes may need to consider the formation of secondary phases, as this phase is non-active and will not contribute to the capacity of LFP. Therefore, the use of nano-C/LFP is a promising strategy for future high-energy density and high-rate capability materials, as they can produce a single phase and stable C/LFP. In addition, it is important to note that such a size-dependent surface phase behaviour may also exist within other olivine phosphate or insulated electrode materials that undergo carbon coating. Sample preparation The LiFePO 4 ingot sample was provided by Phostech Lithium Inc. (Montreal, Canada). There are two reasons for choosing this model material: first, the ingot material is commercially available and commonly used, so the typical behaviours are applicable for other LFP materials. Second, this ingot with a flat, smooth and polished surface is ideal for directly observing and investigating surface chemistry change during carbon coating—for both the bulk olivine phase and secondary intercrystalline phases. Melt casting was performed within an air-tight box furnace under an Ar or N 2 protection in a graphite or alumina crucible between 950 and 1,050 °C. Low-cost various precursors such as iron, LiOH and H 3 PO 4 were used for ingot synthesis. The detailed precursor compositions have been investigated in a previous paper [21] . The small laboratory samples (kg grades) were cooled to room temperature within the box furnace under the protection of an Ar atmosphere. The details of the melt-casting process including experimental details, physical property and electrochemical performance can be found in previous work [22] , [23] . Here, to get a flat surface on the ingot sample, the melt sample was cut into a smaller size using a manual saw, and then the surface was polished using sandpapers (London, 3M Canada) from coarse (Grit 120) to fine grades (Grit 1500). After ultrasonic cleaning in ethanol several times, a LiFePO 4 ingot sample with a clean and flat surface was thus obtained. Powder-based LiFePO 4 samples with different sizes (mm, micro and nano grades) were controlled by ball milling the above LiFePO 4 ingot sample, and detailed experimental process can be obtained in previous papers [24] , [25] . The synthesis technique of LiFePO 4 ingot was also described by Zaghib et al . [20] , [36] , and a high-rate performance of LiFePO 4 was achieved after grinding molten ingot to nanoparticles. In addition, another nano sample, commercial LiFePO 4 powder (Phostech) without carbon coating, was also used in this work. Carbon coating Carbon-coating experiments on ingot samples were performed in a spray-pyrolysis system, which was previously developed for the synthesis of various nanomaterials. In the experiment, alcohol was used as the carbon precursor and argon acted as a carrying and protecting gas. Briefly, the ingot sample with the flat surface up was put in a quartz tube and Ar was introduced into the quartz tube for 20 min to eliminate the air. Subsequently, the furnace was heated, and the carbon-coating process was performed at temperatures ranging from 600 °C to 900 °C for 20 min. After the carbon coating, the coated sample was cooled to room temperature within the furnace still under the protection of the Ar atmosphere. Carbon-coated LiFePO 4 powder samples were prepared by the conventional solid-state method. Lactose (carbon precursor) was firstly dissolved in either isopropyl alcohol or H 2 O, and then various LiFePO 4 powder samples were added to the carbon precursor solution. The suspension was mixed ultrasonically, and was then allowed to evaporate to dryness. The sample was further annealed at 700 °C for 1 h under Ar protection to form carbon-coated samples. Characterization The morphology and microstructure of the samples were characterized using an S-4800 SEM (Hitachi) equipped with an energy-dispersive X-ray microanalysis system and a field-emission gun. X-ray diffraction analyses of the ingot sample was performed using a Bruker D8-Advantage powder diffractometer with Cu K α radiation (1.54056 Å) between 10° and 80° in reflection geometry. Focused ion beam lithography was used for in situ sectioning of the impurity phases, which were imaged and identified by SEM. The slicing process was performed on a LEO (Zeiss) 1540XB FIB/SEM (Western Nanofab., University of Western Ontario), and subsequently the slices were plucked using a nanomanipulator. After the tip of the end effector was folded over and removed from the nanomanipulator rod, the sample could be mounted in the HRTEM sample holder. HRTEM and energy-dispersive X-ray spectroscopy (EDX) analysis at different phases were performed using a JEOL 2010 FEG instrument operating at an accelerating voltage of 200 kV. The diffraction patterns were also recorded using the SAED mode. The P L 3,2 -edge XANES spectra were performed at the Canadian Light Source (CLS) on the Variable Line Spacing Plane Grating Monochromator (VLS PGM) beamline. In situ carbon-coating experiment was performed at Hitachi SEM (S-4800) with a heating carrier designed by Protochips, which enable in situ annealing and real-time observation. Carbon gas (ethylene) was introduced to the sample surface in the SEM chamber to perform carbon coating. Hard X-ray spectroscopic imaging and tomography The transmission X-ray microscopy spectroscopic imaging and nano-tomography with hard X-ray were conducted at beamline X8C, NSLS, Brookhaven National Laboratories (BNL). A field of view of 40 × 40 μm 2 with a 2k × 2k CCD camera was used. A full XANES image series was collected on the FIB sample. Each XANES image series was measured by scanning Fe absorption K-edge from 7,089 to 7,189 eV, with 2 eV step size, and one TXM image at one energy step, which generate 1k × 1k XANES spectra with 2 × 2 binned pixels. Each image was collected with 10 s exposure time. For tomography collection, the data set was collected with 7,120 eV X-rays, using 1,441 projections over an angular range of 180°. The pixel size was 38.9 nm. All the XANES data analysis was carried out using customized program (MatLab, MathWorks, R2011b) developed in house (beamline X8C group, NSLS, BNL). Background normalization was carried first out for TXM images, with a unique background image collected at every energy. With all 1,024 × 1,024 pixels, we can extract the full spectrum (X-ray intensity versus energy) for each pixel. The standard XANES spectra for the reference materials LiFePO 4 (Phostech Lithium Inc.) and new phase were measured at the TXM beamline X8C (NSLS, BNL). The TXM XANES imaging on the reference materials was carried out by using the same condition as used in the XANES imaging for the FIB sample. The tomographic reconstruction was carried out with standard filtered back-projection algorithm. How to cite this article: Wang, J. et al . Size-dependent surface phase change of lithium iron phosphate during carbon coating. Nat. Commun. 5:3415 doi: 10.1038/ncomms4415 (2014).